Enantioselective access to tricyclic tetrahydropyran derivatives by a remote hydrogen bonding mediated intramolecular IEDHDA reaction Inverse-electron-demand-hetero-Diels-Alder reactions of alkenes with α,β-unsaturated keto compounds allow rapid access to the tetrahydropyran ring found in numerous natural products and bioactive molecules. Despite its synthetic interest, catalytic asymmetric versions of this process remain underdeveloped, especially regarding the use of non-activated alkenes reacting with α,β-unsaturated ketone or aldehyde, for which no report can be found in the literature. Herein, we describe the catalytic inverse-electron-demand-hetero-Diels-Alder reactions between neutral alkenes and an α,β-unsaturated ketones or aldehydes to produce a variety of trans-fused [5,6,8] tricyclic structures containing a central, chiral tetrahydropyran ring. This complex transformation, which is achieved using a chiral phosphoric acid, allows for the formation of four stereogenic centers in a single step with high regio-, diastereo- and enantioselectivity (up to 99% ee). Such level of stereocontrol could be achieved by a key remote double hydrogen atom bonding interaction between the linear substrate and the catalyst. Trans-fused [5,6] bicycles containing a tetrahydropyran ring are privileged structural motifs that can be found in numerous natural products and/or bioactive compounds. For example, natural products Englerin A ( 1 ) and Parvifolal A ( 2 ) (Fig. 1a ), which, respectively, exhibit selective cytotoxic activity for renal cancer cell lines and inhibitory activity against sbLOX-1, feature a central trans-fused tetrahydropyranocyclopentane motif A [1] , [2] . The analogous nitrogen atom-containing bicyclic structure—i.e. the octahydropyranopyrrole motif B is also present in a series of synthetic bioactive molecules as exemplified by the tachykinin receptor antagonist 3 and the alpha-1 adrenergic antagonist 4 (Fig. 1b ) [3] , [4] . Despite the importance and the wide occurrence of structural motifs A and B, very little attention has been brought to their enantioselective construction. This situation is in sharp contrast with the numerous efforts made to access the analogous full carbon trans-fused [5,6] hydrindane and tetrahydroindane bicyclic motifs (for selected works involving the synthesis of the challenging trans -hydrindane motif see ref. [5] and for selected studies on the synthesis of the trans -tetrahydroindane motif see ref. [7] ) [5] , [6] , [7] , [8] . Among the various approaches that could be considered to build chiral tetrahydropyran-contained skeletons, the most direct one would most probably consists of implementing an asymmetric inverse-electron-demand hetero-Diels–Alder (IEDHDA) reaction between an alkene and an unsaturated carbonyl electrophile (for selected reviews on asymmetric IEDHDA reactions see ref. [9] ) [9] , [10] , [11] , [12] . Although the intermolecular asymmetric IEDHDA reaction involving electron-rich olefins and α,β-unsaturated carbonyl electrophiles is well documented, non-activated alkene substrates have been less studied in such type of reaction due to their comparatively low reactivity [9] , [10] , [11] , [12] . Fig. 1: Bioactive molecules containing a trans-fused tetrahydropyran bicyclic motif. a Selected bioactive natural products with a trans -fused tetrahydropyranocyclopentane motif. b Selected synthetic bioactive molecules with a trans -fused octahydropyranopyrrole motif. Full size image Previous investigations in this field are summarized in Fig. 2 . Cheng and co-workers initially reported the enantioselective intermolecular Diels–Alder reaction between styrene and β,γ-unsaturated ketone esters catalyzed by a Lewis acid-assisted Brønsted acid complex (Fig. 2a ) [13] . Later, Ishihara and co-workers disclosed that bis(oxazoline)/copper(II) species could promote the enantioselective hetero-Diels–Alder (HDA) reaction of β,γ-unsaturated ketoesters with allyl silanes [14] . In addition, Zhang and co-workers demonstrated that the same β,γ-unsaturated ketoester substrates could react with vinylindoles in the presence of an imidodiphosphoric acid to produce [4 + 2] cycloadducts [15] . More recently, the groups of Rueping and Shi independently reported the formation of chiral chromane derivatives by a Brønsted acid catalyzed IEDHDA reaction between a highly reactive ortho -quinone methide intermediate and styrene [16] , [17] . In comparison, catalytic and asymmetric intramolecular IEDHDA reactions of non-activated alkenes have been far less explored (Fig. 2b ). An early example was reported by the group of Narasaka where an α,β-unsaturated imide reacted with a tri-substituted alkene in the presence of a chiral titanium complex [18] . However, despite its high enantioselectivity, the transformation was found inefficient. Kumaran and co-workers later demonstrated that a chiral copper complex could promote the intramolecular IEDHDA reactions between β,γ-unsaturated ketoesters and tri-substituted neutral olefins, while, very recently, Campagne and co-workers disclosed the intramolecular IEDHDA reaction of α,β-unsaturated acyl imidazole with tri-substituted neutral olefin in the presence of a Pybox/Fe(OTf) 3 complex. Despite being efficient and highly enantioselective, these two transformations featured a very limited scope [19] , [20] . Fig. 2: Previous studies in asymmetric IEDHDA with neutral alkene partners and our approach. a Previous studies on intermolecular asymmetric IEDHDA reactions. b Previous studies on intramolecular asymmetric IEDHDA reactions. c Our approach to asymmetric intramolecular IEDHDA via dual hydrogen bonding interaction. d Access to tricyclic tetrahydropyran derivatives by chiral phosphoric acid catalyzed intramolecular IEDHDA reaction. . Full size image To the best of our knowledge, the use of simple α,β-unsaturated ketones or aldehydes as reaction partners in catalyzed asymmetric intramolecular IEDHA with neutral alkenes has not been reported (a single example of a racemic IEDHA reaction involving an enone and vinylethylene carbonates was recently reported by Li and co-workers) [21] . The reason may be found in the low reactivity of neutral alkenes as nucleophilic component (for selected reviews on neutral alkene-participated asymmetric reactions see ref. [22] , for examples on neutral alkene-participated asymmetric reactions see ref. [25] ) [22] , [23] , [24] , [25] , [26] , [27] , [28] , [29] , [30] , [31] , and the difficulty to find a suitable catalyst being able to efficiently “chelate” the simple α,β-unsaturated ketone or aldehyde electrophile in order to achieve a high facial selectivity. In the synthetic approaches presented above, β,γ-unsaturated ketoesters, unsaturated oxazolidinones and acyl imidazoles were employed to efficiently complex with the metal catalyst (see Fig. 2b ). In this context, we anticipated that such a challenging transformation could potentially be achieved in its intramolecular version by using a chiral Brønsted acid (Fig. 2c ) (for selected reviews on the use of chiral Brønsted acids, see ref. [33] ) [32] , [33] , [34] , [35] , [36] , [37] . In the envisaged scenario, the acid would activate the α,β-unsaturated ketone or aldehyde by hydrogen bonding interaction thus favoring the nucleophilic addition of the neutral alkene (for examples of CPA activating carbonyl reactions see ref. [38] ) [38] , [39] , [40] , [41] , while the enantioselectivity could be generated thanks to the presence of an additional hydrogen bond (HB) donor (HX) present in the substrate. If nucleophilic in nature, this HB donor was however considered as a potential source of side product formation since Michael addition to the α,β-unsaturated keto derivative or ene-cyclization reactions could also be possible under the reaction conditions. In this work, we report the results of our investigations which demonstrated the feasibility of our designed approach using a chiral phosphoric acid to cyclize non-activated alkenes with α,β-unsaturated ketones or aldehydes and a remote hydroxyl group as hydrogen bond donor, to induce the enantiocontroled formation of tricyclic tetrahydropyran derivatives by an IEDHDA—keto acetalization cascade reaction (Fig. 2d ). The transformation is efficient (up to 97% yield), and exhibits excellent enantioselectivities (up to 99% ee) and a broad substrate scope (49 examples). Reaction optimization Our studies started with model substrate ( E )- 5a that possesses a hydroxyl HB donor group and an α,β-unsaturated arylketone as the HB acceptor. 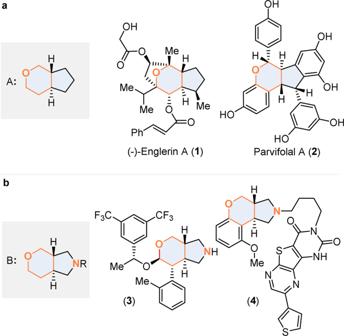Fig. 1: Bioactive molecules containing a trans-fused tetrahydropyran bicyclic motif. aSelected bioactive natural products with atrans-fused tetrahydropyranocyclopentane motif.bSelected synthetic bioactive molecules with atrans-fused octahydropyranopyrrole motif. A series of SPINOL-CPA were evaluated as potential catalysts to achieve the desired transformation (Table 1 ) (for a recent example from our laboratory using CPA see ref. [32] ). The use of phosphoric acid 6a in dichloromethane at 30 °C was rather inefficient. Most of the starting material was found unreacted after 108 h, but, gratifyingly, the formation of the desired product 7a could be observed thus validating our approach. Notably, 7a was produced as a single isomer and no trace of products derived from a competitive Michael addition or an ene-cyclization could be detected. The tricyclic ketal 7a could be isolated in 8% yield and 20% ee (Table 1 , entry 1). Encouraged by this result, a series of SPINOL-CPA were then screened. The enantioselectivity of the reaction could be largely improved and an optimal 95% ee could be obtained using either catalyst 6c or 6d (entries 3 and 7), the latest showing the highest catalytic activity (86% yield). Interestingly, when the catalytic loading was reduced to 5 mol%, the transformation remained robust affording 7a with a lower yield after the same reaction time (67%), but with a very similar level of enantioselectivity (94% ee, entry 9). Employing other solvents in the presence of catalyst 6d was detrimental to both the efficiency and stereoselectivity of the reaction (entries 10–14). Consequently, the use of 20 mol% of catalyst 6d in dichloromethane at 30 °C was retained as optimal conditions to achieve the transformation with high yields and enantioselectivities, and we then investigated the scope of this IEDHDA–keto acetalization cascade reaction. Notably, the IEDHDA reaction of ( Z )- 5a did not proceed at all under the optimal reaction conditions. Table 1 Optimization of the reaction conditions a . Full size table Scope of substrates The effect of substitution on both the alkene and α,β-unsaturated ketone was surveyed. The results are shown in Fig. 3a . As for the alkene part, groups of various electronic nature were tolerated on the phenyl ring substituent R 1 : tri-substituted alkene derivatives 5a–g led to the formation of the corresponding tricyclic products 7a – g in moderate to high yields (50–95%) and with excellent enantioselectivities (90–96% ee). The position of the substituent on the aromatic ring was shown to exert negligible influence on the facial selectivity of this reaction despite the fact that an ortho -MeO substituent led to reduced yield in product when compared to the analogous meta-substituted substrate (compare 7e and 7f ). The presence of a substituent at position ortho may possibly alter the reactivity of the alkene partner by reducing its conjugation with the aromatic ring and/or generating unfavorable steric constraints close to the reaction centers. It is noteworthy that the transformation was not limited to the use of aryl-substituted alkenes. An alkyl group, such as a simple methyl was also compatible and for instance substrate 5h could be converted into the IEDHDA product 7h with an excellent ee value of 93%. The yield of the reaction was however more moderate (40%). The substitution pattern of the α,β-unsaturated ketone moiety was then investigated with substrates 5i–q . The studies showed that in the presence of electron-rich aromatic groups, the desired tricyclic products 7i – m could be obtained in good yields (69–95%) and with high enantioselectivities (89–98% ee). The reaction also tolerated the presence of a heterocyclic ring as exemplified by the efficient and highly selective conversion of substrates 5n–q , that possess a substituted thiophene ring, into products 7n–q . The reaction could also be performed with non-aromatic R 2 groups. An alkyl substituent such as a methyl group or a simple hydrogen atom was fully compatible: the corresponding substrates 5r and 5s were converted into products 7r and 7s with good yields (74% and 91%) and excellent enantiocontrol (91% ee and 95%ee). The transformation could also be extended to the formation of [6-6-8] tricyclic structures: piperidine derivative 7t was formed for instance in 63% yield and with excellent enantioselectivity (97% ee). The relative and absolute configurations of the tricyclic ketals shown in Fig. 3a were deduced by analogy with the stereochemistry of 7e , which was unambiguously assigned as ( R , S , R, R ) by X-ray diffraction analysis (see Supplementary Fig. 2 for more details). To further extend the diversity of products that could be produced, we also wanted to evaluate if the replacement of the NTs moiety by a carbon-based group would alter the efficiency of the process. Fig. 3: Scope of the reaction with α,β-unsaturated ketones as the HB acceptor. a Variation of substituent on both the alkene (R 1 ) and the α,β-unsaturated ketone (R 2 ) for substrates with an tosylamide linker. b Variation of substituent R on the α,β-unsaturated ketone for substrates possessing an all carbon-linker. Reactions were performed with 30 mg of susbtrate 5a–t or 8a–n and 4 Å MS (60 mg) in the presence of catalyst 6d (20 mol%) at 30 °C in 1.0 mL DCM for 48–60 h. Isolated yields are given; only a single stereoisomer was isolated (d.r. > 20:1); ee were measured by chiral HPLC analysis. Full size image Gratifyingly, under the same optimal reaction condition, dibenzylmalonate derivative 8a could be similarly converted into 9a which was isolated in 94% yield and with 96% ee, thus demonstrating the wide applicability of the process (Fig. 3b ). A series of substrate 8b–n featuring the same malonate linker but variously substituted α,β-unsaturated ketones were then reacted (Fig. 3b ). High yields and enantioselectivities (up to 96% yield and 99% ee) could be achieved with substrates 8b – j which possess either electron-rich or poor aromatic substituents. Importantly, enones substituted by an alkyl group were suitable substrates as shown by the formation of products 9k – n . While enantioselectivities remain uniformly high (97–99% ee) whatever the nature of the alkyl group, reduced yields were obtained in the case of cyclic alkyl substituents ( 9m and 9n ). This relative loss of efficiency was tentatively attributed to the lower stability of the ketal moiety in 9m - n , which were observed to be more prone to hydrolysis under the acidic reaction conditions. For such types of organocatalytic transformations, the reactivity of α,β-unsaturated aldehydes is generally quite different from that of α,β-unsaturated ketones. However, in the present case, when substrate 10a was subjected to the optimized reaction conditions, the tricycle product 11a could also be obtained in a good yield and with an excellent ee value (95% yield, 95% ee, Fig. 4 ). This reactivity could be generalized as attested by the results obtained with substrates 10b – p bearing various malonate linkers and/or alkene substituents (Fig. 4 ). The nature of the malonate substituents on 10a–j had negligible influence on the enantiocontrol (93–95% ee) and yields in tricyclic products 11a – j were generally high (73–95%). A similar trend was observed when the nature of the aromatic substituent on the alkene was varied: slightly lower yields (65–79%) were obtained as compared to the reaction of 10a , while the enantioselectivity remained high (91–99%ee, 11k–p ). The absolute configuration of product 11a was unambiguously confirmed as ( R , S , R , R ) by X-ray analysis (Fig. 4 , see Supplementary Fig. 3 for more details). Fig. 4: Scope of the reaction with α,β-unsaturated aldehyde as the HB acceptor. Reactions were performed with 30 mg of substrate 10a–p and 4 Å MS (60 mg) in the presence of catalyst 6d (20% mol) at 30 °C in 1.0 mL DCM for 60 h. Isolated yields are given; only a single stereoisomer was isolated (d.r. > 20:1); ee were measured by chiral HPLC analysis. Full size image Product derivatization To further demonstrate the synthetic usefulness of the catalytic transformation thus developed, a series of post-transformations were performed (Fig. 5 ). The ketal motif in 7o could be reduced to generate the octahydropyranopyrrole 12 in 71% yield, 7:1 d.r. and without erosion of enantioselectivity (97% ee). The eight-membered cyclic ether in structure 7h could alternatively be oxidized at room temperate to furnish lactone 13 [42] . A subsequent alcoholysis step led to chiral pyrrolidine derivative 14 that contains three contiguous stereogenic centers. The ketal moiety in product 11a could undergo an efficient stereoselective allylation reaction to produce the bicyclic product 15 in 68% yield. Finally, it was shown that the same tricyclic compound 11a could be hydrogenated to quantitatively afford the dicarboxylic acid 16 , which in turn could be transformed into monoacid 17 with the generation of a new stereogenic center. This selection of classical functional group conversions demonstrates the synthetic potential of the present asymmetric catalytic IEDHDA reaction to generate structural diversity. Fig. 5: Post-transformations of IEDHDA products. Reaction conditions: a DIBAL-H, CH 2 Cl 2 , 0 °C, 71% (d.r. = 7:1), 97%ee. b RuCl 3 , NaIO 4 , CH 3 CN/CHCl 3 /H 2 O, RT, 45%, 93%ee. c K 2 CO 3 , MeOH, RT, 65%, 93%ee. d Allyltrimethylsilane, SnCl 4 , −30 °C to RT, CH 2 Cl 2 , 68%, 95%ee. e Pd/H 2 , MeOH, quant. ; f Pyridine, reflux, 78%, 95%ee. Full size image Mechanistic studies We then worked at determining the mechanism of the reaction and rationalizing the observed high enantioinduction. We first studied the HB donor role of the hydroxyl group in the process (Fig. 6a ). To this purpose, the TBS-protected substrate 18 , derivative from model substrate 5a , was prepared and subjected to the optimal reaction conditions. The IEDHDA dihydropyran product 19 was formed in a moderate 41% yield that was attributed to the tendency of 19 to be hydrolyzed under the acidic reaction conditions as well as during the purification step by flash column chromatography. Most importantly, 19 was produced with a significantly reduced 49% ee, as compared to the formation compound 7a from the parent free OH substrate 5a (86% yield, 95% ee, see Table 1 , entry 7). This result suggests that the hydroxyl group on 5a may function not only as the nucleophile in the cascade process leading to the formation of the ketal product, but also as a remote hydrogen donor to enhance the interaction between substrate 5a and catalyst 6d , and thus improving the facial selectivity in the process. If catalyst 6d allows the IEDHDA reaction to take place through a dual hydrogen bonding interaction, the strength of the interaction between the substrate and the catalyst and the consequent spatial organization should logically be affected by the distance between the hydroxyl moiety and carbonyl group. Fig. 6: Probing the HB interaction. 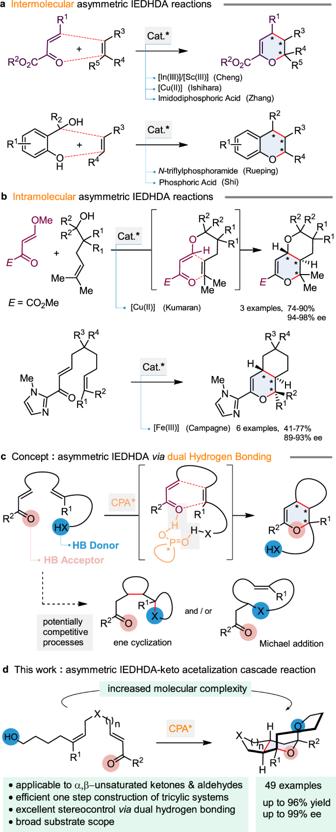Fig. 2: Previous studies in asymmetric IEDHDA with neutral alkene partners and our approach. aPrevious studies on intermolecular asymmetric IEDHDA reactions.bPrevious studies on intramolecular asymmetric IEDHDA reactions.cOur approach to asymmetric intramolecular IEDHDA via dual hydrogen bonding interaction.dAccess to tricyclic tetrahydropyran derivatives by chiral phosphoric acid catalyzed intramolecular IEDHDA reaction. . a IEDHDA reaction with a substrate lacking the HB donor. b Effect of the HB donor-alkene linker size on the enantiocontrol. Full size image Based on this speculation, a series of substrate 5u–w possessing alkene/hydroxyl linkers of various sizes were synthesized and reacted under the standard reaction conditions. The IEDHDA reactions with 5u–w took place and could provide the corresponding tricyclic products 7u-w as well as the by-products 7u ′– 7w ′ due to the competitively intramolecular Michael addition of the hydroxyl group to the enone moiety and side product N , O -acetal 7w ″ in the case of 5w as well. The results obtained (Fig. 6b ) clearly show a decrease of the ee values when the linker is shortened. Substrates 5v and 5w afforded the desired tricyclic product 7v and 7w but in moderate yield (respectively, 60% and 30% yield) and both with a 50% ee which appeared to be the same enantiocontrol obtained for the conversion of TBS-ether 18 into 19 . These results suggest that a dual hydrogen bonding interaction may not be in play for the conversion of 5v and 5w due to an unfavorable spatial distance between the hydroxyl HB donor and the carbonyl HB acceptor. In these cases, the lack of structural flexibility in the substrates may lead to the inability of catalyst 6d to properly “coordinate” to 5v or 5w in a dual manner. On the basis of these experiments and by taking into account the absolute configuration of the tricyclic products obtained, we proposed the catalytic mechanism as shown in Fig. 7 . In this model, the terminal hydroxyl group in 5a would interact with the P = O functionality of catalyst 6d , while the P–OH moiety would electrophilically activate the carbonyl group in 5a . Both HB interactions between 5a and 6d should be synergistically involved to induce the IEDHDA reaction via a spatially well-organized transition state such as TS1-1 . The resulting dihydropyran intermediate 20 would be further activated by the acidic catalyst to promote the ketalization step leading to 7a via transition state TS2 . From a selectivity point of view, it is proposed that the Si face of the trisubstituted alkene could be preferentially reacted with the Si face of the conjugated enone (as shown in TS1-1 ). This mechanism was supported by density-functional theory (DFT) calculations performed on substrate 5a (see Supplementary Discussion for more details). The computational studies showed TS1-1 to be energetically more favorable than TS1-1 ′ by 2.6 kcal/mol, a value in agreement with the level of enantioselectivity experimentally observed. Interestingly, the formation of the dihydropyran moiety was calculated to proceed in a stepwise manner. The cyclization process would be initiated by the formation of the C 1 –C 2 bond via TS1-1 , a step that would be rate determining. A subsequent facile C 3 –O bond formation (1.5 kcal/mol) would deliver intermediate 20 . 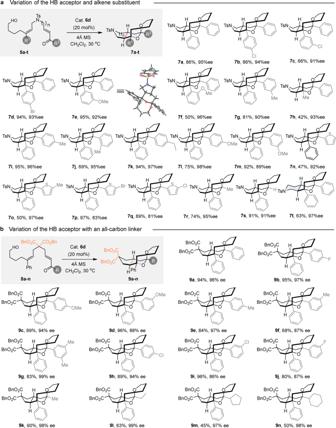Fig. 3: Scope of the reaction with α,β-unsaturated ketones as the HB acceptor. aVariation of substituent on both the alkene (R1) and the α,β-unsaturated ketone (R2) for substrates with an tosylamide linker.bVariation of substituent R on the α,β-unsaturated ketone for substrates possessing an all carbon-linker. Reactions were performed with 30 mg of susbtrate5a–tor8a–nand 4 Å MS (60 mg) in the presence of catalyst6d(20 mol%) at 30 °C in 1.0 mL DCM for 48–60 h. Isolated yields are given; only a single stereoisomer was isolated (d.r. > 20:1); ee were measured by chiral HPLC analysis. Fig. 7: Mechanistic proposal. a Proposed catalytic cycle. b Transition state model of stereocontrol. Full size image In conclusion, we have developed a chiral phosphoric acid-promoted enantioselective IEDHDA-keto-acetalization cascade transformation that involves the initial reaction of either α,β-unsaturated ketones or aldehydes with non-activated alkenes to ultimately produce trans-fused octahydropyranopyrrole and trans-fused tetrahydropyrano-cyclopentane tricyclic frameworks. The transformation was shown highly enantioselective and could be applied to a variety of substrates. The design of the remote dual HB interaction was key to achieving high chiral induction in this challenging transformation. Application of this concept to the development of other organocatalytic reactions is currently underway in our laboratory. General procedures for the IEDHDA reactions Substrate 5a–t , 8a–n or 10a–p (30 mg, 1.0 eq.) 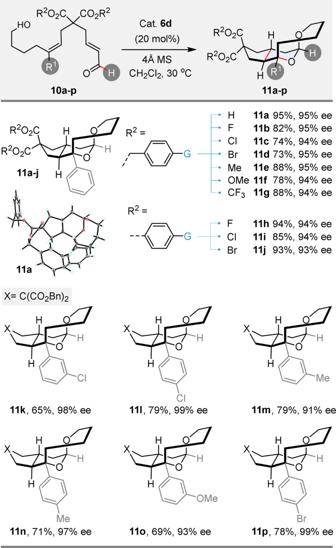Fig. 4: Scope of the reaction with α,β-unsaturated aldehyde as the HB acceptor. Reactions were performed with 30 mg of substrate10a–pand 4 Å MS (60 mg) in the presence of catalyst6d(20% mol) at 30 °C in 1.0 mL DCM for 60 h. Isolated yields are given; only a single stereoisomer was isolated (d.r. > 20:1); ee were measured by chiral HPLC analysis. was dissolved in anhydrous DCM (1.0 ml), then 4 Å molecular sieves (60.0 mg) and catalyst 6d (0.2 eq.) were added. The reaction mixture was sealed and stirred at 30 o C and monitored by TLC (generally for 48–60 h). 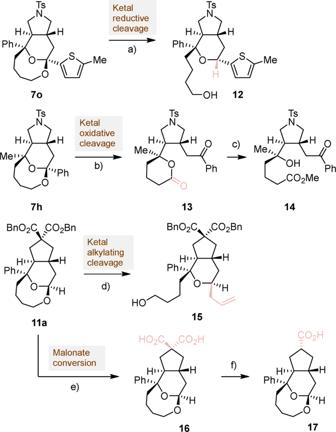Fig. 5: Post-transformations of IEDHDA products. Reaction conditions:aDIBAL-H, CH2Cl2, 0 °C, 71% (d.r. = 7:1), 97%ee.bRuCl3, NaIO4, CH3CN/CHCl3/H2O, RT, 45%, 93%ee.cK2CO3, MeOH, RT, 65%, 93%ee.dAllyltrimethylsilane, SnCl4, −30 °C to RT, CH2Cl2, 68%, 95%ee.ePd/H2, MeOH, quant.;fPyridine, reflux, 78%, 95%ee. 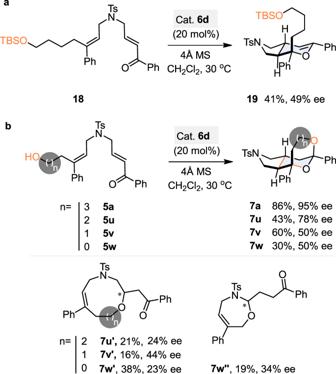Fig. 6: Probing the HB interaction. aIEDHDA reaction with a substrate lacking the HB donor.bEffect of the HB donor-alkene linker size on the enantiocontrol. 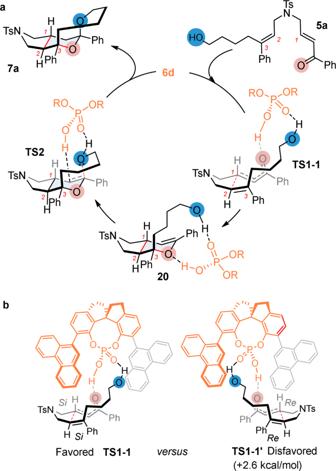Fig. 7: Mechanistic proposal. aProposed catalytic cycle.bTransition state model of stereocontrol. When the reaction was completed, the mixture was directly purified by silica gel column to afford products 7a–t , 9a–n , or 11a–p, respectively.